Condensin I associates with structural and gene regulatory regions in vertebrate chromosomes The condensin complex is essential for correct packaging and segregation of chromosomes during mitosis and meiosis in all eukaryotes. To date, the genome-wide location and the nature of condensin-binding sites have remained elusive in vertebrates. Here we report the genome-wide map of condensin I in chicken DT40 cells. Unexpectedly, we find that condensin I binds predominantly to promoter sequences in mitotic cells. We also find a striking enrichment at both centromeres and telomeres, highlighting the importance of the complex in chromosome segregation. Taken together, the results show that condensin I is largely absent from heterochromatic regions. This map of the condensin I binding sites on the chicken genome reveals that patterns of condensin distribution on chromosomes are conserved from prokaryotes, through yeasts to vertebrates. Thus in three kingdoms of life, condensin is enriched on promoters of actively transcribed genes and at loci important for chromosome segregation. The structural maintenance of chromosome (SMC) proteins are essential for chromosome segregation in species ranging from prokaryotes to humans. SMC proteins are ABC ATPases, capable of altering DNA topology through cycles of ATP binding and hydrolysis [1] , [2] . SMC proteins bind in pairs, and six distinct SMCs exist in eukaryotes that form three complexes. Although SMCs are structurally similar, they have diverse functions, with SMC1/3 (cohesin) involved in sister chromatid cohesion and gene regulation, SMC5/6 in DNA repair and SMC2/4 (condensin) in chromosome architecture [3] , [4] . SMC proteins phylogenetically predate the histones, and are essential for control of diverse aspects of the cell cycle through their ability to modify and modulate chromatin. They are increasingly touted as global genome organizers due to their diverse roles in a number of essential cell cycle functions [5] . A fundamental advance in understanding chromosome packaging was made with the discovery of condensin, a highly conserved pentameric complex assembled around two SMC proteins. Condensin is an ancient protein complex conserved from prokaryotes to eukaryotes [6] . There are two forms of condensin in vertebrates: condensins I and II. Both are composed of the SMC2 and SMC4 ATPases plus three auxiliary subunits called condensin-associated proteins (CAP): CAP-G, CAP-D2 and CAP-H for condensin I; CAP-G2, CAP-D3 and CAP-H2 for condensin II [3] , [7] , [8] . Studies in a variety of organisms have shown that the condensin complex has a crucial role in the formation and segregation of structurally stable mitotic chromosomes into daughter nuclei [5] , [9] , [10] . In vertebrates, condensin I is confined to the cytoplasm during interphase and loaded onto the chromosomes at the end of prophase after nuclear envelope break down (NEBD) [11] , [12] . By contrast, condensin II localizes to the DNA in both interphase and mitosis. Condensin localization in vertebrates has been studied intensively in fixed cells using condensin antibodies, and in vivo with GFP-tagged condensin subunits [11] , [12] , [13] , [14] . However, to date, condensin-binding sites in the vertebrate genome have remained elusive. Some clues to where condensin might bind in vertebrates have been provided by genome-wide studies in bacteria and yeast. The prokaryotic condensin-like SMC homodimer found in B. subtilis is loaded via ParB/Spo0J onto centromere-like sequences called par S [15] , [16] . The binding sites are close to the DNA replication origins, suggesting condensin might help to compact the newly replicated DNA in readiness for chromosome segregation [15] . Genome-wide condensin maps in S. cerevisiae and S. pombe show that condensin binds to discrete sites in the genome [17] , [18] . Yeast condensin is recruited via the cohesin loader Scc2–Scc4, and is enriched at centromeres and along the chromosome arms at highly transcribed tRNA and rRNA genes [17] . In addition to its established role in chromosome segregation, condensin has a less-understood role in regulating gene expression. In yeast, condensin modulates rDNA arrangement in the nucleus and is responsible for maintaining silent chromatin domains in the genome [19] . In D. melanogaster , the condensin I subunit CAP-G both enhances and suppresses position effect variegation (PEV), whereas CAP-D3/condensin II mutants suppress PEV [20] . Other studies in D. melanogaster suggest that CAP-D3 directly interacts with the retinoblastoma protein RBF1, regulating the expression of genes of the innate immune system [21] , [22] . In human cells, protein phosphatase 2A (PP2A) recruited by HSF2 to the hsp70 promoter inactivates condensin I, and results in decreased compaction of the promoter region in mitosis [23] , [24] . This is termed bookmarking, and leads to increased transcription of the bookmarked genes in the following G1 (refs 24 , 25 ). To address the role of condensin I in vertebrates, we have used a method analogous to ChIP-seq to create the first genome-wide map of condensin I-associated DNA in chicken DT40 lymphoma B cells. Our genome-wide map of condensin I is complemented by direct functional analysis using qRT–PCR of RNA isolated from CAP-H/condensin I knockout (KO) cells in G1 phase. Despite the difference in genome size and organization between bacteria, yeast and vertebrates, patterns of condensin I binding are similar. In all, condensin is highly enriched on tRNA and rRNA genes and at centromeres. Chicken condensin I is also enriched at promoters of RNA polymerase II-driven genes and at non-coding RNA genes such as tRNA and rRNA genes. Condensin I binds at a number non-genic DNAs including centromere and telomere sequences. These results show that condensin I predominantly associates with loci that have some degree of transcriptional activity. Consistent with a putative bookmarking role of condensin I, we found that its removal affects the transcription of a number of genes during the following G1 phase. Genome-wide distribution of condensin I To determine where condensin I is located along the vertebrate chicken (DT40) genome during mitosis we utilized genetic knockouts for CAP-H (representing condensin I only) and SMC2 (representing both condensin I and II) rescued with streptavidin-binding peptide (SBP) affinity-tagged transgenes ( Supplementary Fig. S1 ). Both transgenes completely rescued their cognate knockout cells, producing SBP staining characteristic of the axial localization of condensin I during mitosis and showing essentially complete overlap with another condensin I complex subunit CAP-D2 ( Supplementary Fig. S1A ). Importantly for subsequent analyses, the level of the SBP-tagged rescuing protein was similar to the endogenous level for both wild-type SMC2 and CAP-H ( Supplementary Fig. S1B ). Live cell imaging of CAP-H–GFP–SBP ( Supplementary Fig. S1C ) revealed condensin I in chicken DT40 cells to be excluded from the nucleus in interphase, to accumulate on chromatin following NEBD and then to disappear from chromatin at the end of telophase. This is consistent with vertebrate wild-type condensin I localization in other reports [11] , [12] . The SBP tag shows remarkable purification for the condensin complex in both uncrosslinked and importantly crosslinked samples ( Supplementary Fig. S2 ), which is key to our downstream sequencing applications. To create a genome-wide map of condensin I-binding sites, DNA bound to the condensin I subunits SMC2 and CAP-H was sequenced as well as the respective input DNAs. We will refer to this analysis as Chromatin Affinity Purification-sequencing (ChAP-seq) as pulldowns were performed using SBP-tagged proteins and streptavidin beads. This is therefore analogous to ChIP-seq, where antibodies are used for chromatin immunoprecipitation. As condensin I is only present on DNA during mitosis, only mitotically blocked SMC2–SBP and CAP-H–GFP–SBP were processed. Using 24–36 million 50-bp single-end reads ( Supplementary Table S1 ), we identified multiple regions of condensin I enrichment in the chicken genome. Duplicate sequences were removed in this analysis in order to minimize PCR bias. Model-based Analysis for ChIP-seq (MACS), a model-based peak-calling program [26] , identified 6,474 SMC2 and 4,369 CAP-H-specific peaks in DT40 cells ( Fig. 1a ), and identified 2,140 regions shared between them which includes multiple shared peaks. The widths and intervals between the peaks vary widely. The average peak width for SMC2 was 1,442 bp (ranging from 437 to 40,356 bp). The average for CAP-H was 2,849 bp (ranging from 306 to 30,276 bp). The average distance between peaks was 172 kb (3 bp to 12,677 kb) for SMC2 and 257 kb (2 bp to 8,237 kb) for CAP-H, taking into account the 1.2-Gb size of the chicken genome. 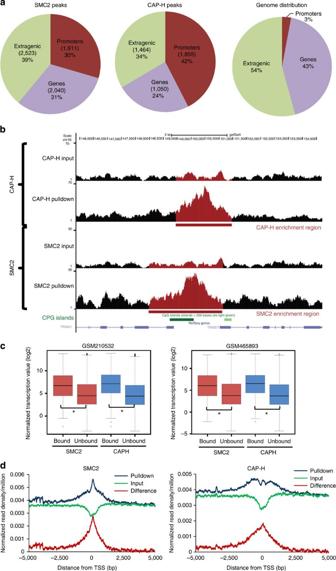Figure 1: Enrichment of chicken condensin I complexes at promoter regions in mitotic chromosomes. (a) The landscape of SMC2 and CAP-H enrichment peak distribution at genomic features including promoters, genes and extragenic sequences. The data show that the majority of enrichment regions for SMC2 or CAP-H are located in promoter regions. Enrichment peaks of SMC2 and CAP-H were independently called with respect to their input, and counted in these features. The numbers in the brackets are the raw peak number for each feature. Genomic distribution indicates the base-coverage of each feature in the chicken genome (galGal4). (b) CAP-H and SMC2 pulldown enrichment to input in the promoter regions for the bidirectionalTRIM27andTRIM41genes. The coordinate of this view is chr16:145,376-154,212 of chicken galGal4 genome. (c) Condensin I binds actively transcribed genes. Transcription levels of NCBI RefSeq genes from wild-type chicken DT40 cells were obtained from two independent Affymetrix data sets in Genome Expression Omnibus (GSM210532, GSM465893), and the transcription of SMC2 (1,531) or CAP-H-peak-bound genes (1,612) and those without condensin peaks (9,137 and 9,056, respectively) were compared. Transcription levels of 10,668 RefSeq genes of total 17,148 were available from the data sets.yaxis represents normalized transcription values in log2. Note bothP-values between condensin-bound and unbound genes (denoted by asterisk) in two independent Affymetrix data sets are <2.2 × 10−6as calculated by Wilcoxon Rank Sum test. (d) High density of SMC2 and CAP-H sequence tags at TSS of all RefSeq genes in the chicken galGal4 genome assembly. Pulldown of SMC2 and CAP-H at (TSS) in the chicken genome is highly enriched compared to the input. Thexaxis is the distance from the (TSS) up to 5 kb up and downstream andyaxis is the normalized sequence read density. SMC2 or CAP-H pulldowns and input are shown as blue and green, respectively, and the read number difference between these two is in red. Figure 1: Enrichment of chicken condensin I complexes at promoter regions in mitotic chromosomes. ( a ) The landscape of SMC2 and CAP-H enrichment peak distribution at genomic features including promoters, genes and extragenic sequences. The data show that the majority of enrichment regions for SMC2 or CAP-H are located in promoter regions. Enrichment peaks of SMC2 and CAP-H were independently called with respect to their input, and counted in these features. The numbers in the brackets are the raw peak number for each feature. Genomic distribution indicates the base-coverage of each feature in the chicken genome (galGal4). ( b ) CAP-H and SMC2 pulldown enrichment to input in the promoter regions for the bidirectional TRIM27 and TRIM41 genes. The coordinate of this view is chr16:145,376-154,212 of chicken galGal4 genome. ( c ) Condensin I binds actively transcribed genes. Transcription levels of NCBI RefSeq genes from wild-type chicken DT40 cells were obtained from two independent Affymetrix data sets in Genome Expression Omnibus (GSM210532, GSM465893), and the transcription of SMC2 (1,531) or CAP-H-peak-bound genes (1,612) and those without condensin peaks (9,137 and 9,056, respectively) were compared. Transcription levels of 10,668 RefSeq genes of total 17,148 were available from the data sets. y axis represents normalized transcription values in log2. Note both P -values between condensin-bound and unbound genes (denoted by asterisk) in two independent Affymetrix data sets are <2.2 × 10 −6 as calculated by Wilcoxon Rank Sum test. ( d ) High density of SMC2 and CAP-H sequence tags at TSS of all RefSeq genes in the chicken galGal4 genome assembly. Pulldown of SMC2 and CAP-H at (TSS) in the chicken genome is highly enriched compared to the input. The x axis is the distance from the (TSS) up to 5 kb up and downstream and y axis is the normalized sequence read density. SMC2 or CAP-H pulldowns and input are shown as blue and green, respectively, and the read number difference between these two is in red. Full size image To further analyse the data, we categorized the peaks from both SMC2 and CAP-H into those occupying promoters, genes (NCBI RefSeq genes and all non-coding RNA genes) and extragenic regions. Distributions of condensin I and total condensin-binding sites were broadly similar ( Fig. 1a ). We defined promoter regions as 2 kb upstream from transcription start sites (TSSs) of all RefSeqGene project including protein-coding and non-coding genes available from NCBI RNA reference sequences [27] . Our analysis showed enrichment of condensin I at promoters with 30% of SMC2 and 42% of CAP-H peaks in these regions ( Fig. 1a ). Despite attracting 30% and 42% of SMC2 and CAP-H respectively, promoters represent only 3% of the chicken genome ( Fig. 1a ). Remarkably, the smallest proportion of condensin-binding sites corresponding to 31% of SMC2 and 24% of CAP-H were located in the bodies of transcribed genes (excluding promoters), which we defined as the regions between the TSSs to the end of the 3′ UTR of RefSeq genes comprising 43% of the chicken genome ( Fig. 1a ). These results suggest that condensin prefers to associate with regions of ‘open’ chromatin. Although non-coding RNA genes, including tRNA and rRNA genes, comprise only 0.0008 of the chicken genome [28] , [29] , 1.4% for SMC2 and 2.7% for CAP-H peaks were localized in the non-coding RNA genes. About 39% of SMC2 peaks were extragenic compared with 34% for CAP-H. Condensin I is enriched at promoters of active genes To more precisely assess the overall enrichment of condensin I at promoters, we identified 1,247 genes from a total of 17,148 in chicken genome having both SMC2 (2,335) and CAP-H (2,360) associated with their promoters. Of these, 1,058 (~84%) are associated with CpG islands, compared with only ~52% of the total promoters associated with CpG islands in the chicken genome ( Supplementary Fig. S3 ). An example of condensin I enrichment on a CpG island promoter for two bidirectional genes ( TRIM27 and TRIM41 ) is presented in Fig. 1b as a UCSC genome browser snapshot. To determine the activity of condensin-bound genes, transcriptions of condensin-bound and unbound RefSeq genes were analysed using DT40 expression database. Affymetrix DT40 expression array analysis revealed clearly that condensin binds preferentially to highly transcribed genes ( Fig. 1c ). This is in agreement with the mapping of bacterial SMC and also cohesin and condensin in yeast suggesting a strongly conserved evolutionary feature amongst condensin-like proteins [15] , [30] . Furthermore, gene ontology analysis shows that the most significant functional roles of the condensin-associated genes are in chromosome and genome organization as well as in cellular and metabolic process ( Supplementary Table S2 ). In addition to showing an accumulation in more distal gene regions, our data reveal that condensin tends to accumulate at the TSSs of RefSeq genes. We analysed the total read density for SMC2 and CAP-H at the TSS for all chicken RefSeq genes. Total reads for SMC2 and CAP-H showed a dramatic increase over the TSS ( Fig. 1d ). If the TSS analysis is demarked between high and low expressed genes as determined by Affymetrix gene expression analysis, condensin I again peaks over the TSS for highly expressed genes but is relatively lower for more weakly expressed genes ( Supplementary Fig. S4 ). This further suggests that the genomic distribution of condensin is correlated with open chromatin and provides compelling evidence that condensin I preferentially binds to the promoters of actively transcribed genes. Condensin I enrichment at non-coding RNA genes Condensin I subunits were highly enriched at loci containing tRNA and rRNA genes. For example, SMC2 and CAP-H are enriched greater than twofold compared with the input in >70% (198 and 197 genes for SMC2 and CAP-H, respectively) of the 279 tRNA genes annotated in the chicken genome [28] , and the majority of them (173 genes) are both SMC2 and CAP-H enriched ( Fig. 2a , Supplementary Fig. S5 ). An average enrichment of 4.08- and 4.67-fold for SMC2 and CAP-H, respectively, was found for all tRNA genes. An example of a condensin I peak encompassing a number of tRNA genes is presented in Fig. 2b . As the tRNA genes are short (71–115 bp) and frequently overlap with CpG islands, we further separated tRNA genes that overlap CpG islands (94 tRNA genes) from those that do not (185 tRNA genes). We found that SMC2 and CAP-H are enriched on average 5.6- and 7.2-fold over input, respectively, on tRNA genes that overlap with CpG islands but only about twofold where tRNA genes do not overlap CpG islands ( Fig. 2c ). This suggests that CpG islands and tRNA genes have additive effects on condensin I binding, and that CpG islands are not a prerequisite for condensin I enrichment at tRNA genes. 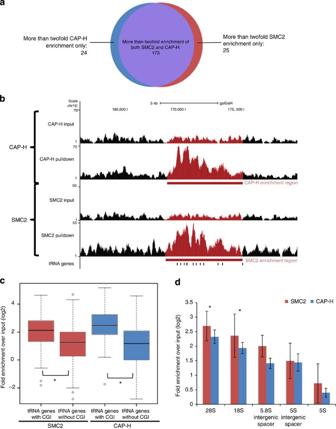Figure 2: Condensin I is abundant in non-coding RNA genes of chicken DT40 cells. (a) Venn diagram showing a large overlap between tRNA genes having greater than two-fold SMC2 or CAP-H enrichment over the input (198 and 197 genes for SMC2 and CAP-H, respectively, of total 279 tRNA genes). The majority of those SMC2 and CAP-H enriched genes overlap (173 genes). The enrichment is measured by total sequence read counts of SMC2 or CAP-H over all known tRNAs. (b) An example of CAP-H and SMC2 pulldown enrichment to the input over a tRNA cluster is shown in the UCSC genome browser snapshot. The coordinate is chr16:161,127-179,974 of galGal4. (c) Box plots of SMC2 and CAP-H enrichment to input in tRNA genes with or without overlapping CpG islands (94 and 185 genes, respectively). Both SMC2 and CAP-H enrichments in the tRNA genes with CpG islands are more prominent (average 5.6- and 7.2-fold for SMC2 and CAP-H, respectively) compared with tRNA genes without a CpG island (average about two-fold for both SMC2 and CAP-H). The difference between these two groups is significant withP-values of 1.2 × 10−8for SMC2 and 4.0 × 10−14for CAP-H (denoted by asterisk) calculated by Wilcoxon Rank Sum test. (d) A bar plot for SMC2 and CAP-H pulldown enrichment to input aligned in the consensus rRNA gene sequences of 28S, 18S, 5.8S intergenic spacer, 5S intergenic spacer and 5S. Significant enrichment of SMC2 and CAP-H relative to input is observed in 28S and 18S rRNA gene sequences having adjustedP-values of 7.34 × 10−4and 5.99 × 10−3, respectively (denoted by asterisk;n=5 as for both SMC2 and CAP-H). Error bars represent standard errors.P-values were calculated using edgeR exact test with Benjamini–Hochberg FDR adjustment31. Figure 2: Condensin I is abundant in non-coding RNA genes of chicken DT40 cells. ( a ) Venn diagram showing a large overlap between tRNA genes having greater than two-fold SMC2 or CAP-H enrichment over the input (198 and 197 genes for SMC2 and CAP-H, respectively, of total 279 tRNA genes). The majority of those SMC2 and CAP-H enriched genes overlap (173 genes). The enrichment is measured by total sequence read counts of SMC2 or CAP-H over all known tRNAs. ( b ) An example of CAP-H and SMC2 pulldown enrichment to the input over a tRNA cluster is shown in the UCSC genome browser snapshot. The coordinate is chr16:161,127-179,974 of galGal4. ( c ) Box plots of SMC2 and CAP-H enrichment to input in tRNA genes with or without overlapping CpG islands (94 and 185 genes, respectively). Both SMC2 and CAP-H enrichments in the tRNA genes with CpG islands are more prominent (average 5.6- and 7.2-fold for SMC2 and CAP-H, respectively) compared with tRNA genes without a CpG island (average about two-fold for both SMC2 and CAP-H). The difference between these two groups is significant with P -values of 1.2 × 10 −8 for SMC2 and 4.0 × 10 −14 for CAP-H (denoted by asterisk) calculated by Wilcoxon Rank Sum test. ( d ) A bar plot for SMC2 and CAP-H pulldown enrichment to input aligned in the consensus rRNA gene sequences of 28S, 18S, 5.8S intergenic spacer, 5S intergenic spacer and 5S. Significant enrichment of SMC2 and CAP-H relative to input is observed in 28S and 18S rRNA gene sequences having adjusted P -values of 7.34 × 10 −4 and 5.99 × 10 −3 , respectively (denoted by asterisk; n =5 as for both SMC2 and CAP-H). Error bars represent standard errors. P -values were calculated using edgeR exact test with Benjamini–Hochberg FDR adjustment [31] . Full size image SMC2 and CAP-H were also enriched on rRNA genes. This enrichment was most significant on the 28S and 18S rRNA genes at fourfold with adjusted P -values of 7.34 × 10 −4 and 5.99 × 10 −3 (calculated using edgeR exact test [31] ), respectively, whereas only a marginal enrichment was found on 5S genes ( Fig. 2d , Supplementary Figs S6 and S7 ). It is important to note that tRNA and rRNA genes were also sites of enriched condensin binding in yeast [17] , [18] and bacteria [15] . It thus appears that patterns of condensin binding are conserved between bacteria, yeast and vertebrates despite the differences in genome complexity and organization. Centromeric enrichment of condensin I Most chicken centromeres are made up of tandemly repeated satellite DNA; however, the centromeres of chromosomes 5, 27 and Z are composed of unique-sequence DNA, which has been fully sequenced [32] . This allows for a specificity of ChAP-seq mapping that is not possible with other highly repetitive vertebrate centromeres. Total condensin and condensin I were dense at centromeric regions of chromosomes 5, 27 and Z, as judged by their overlap with areas previously shown to bind the centromeric histone H3 variant, CENP-A, the signature mark for all active centromeres ( Fig. 3a–c , Supplementary Fig. S8A ) [32] . The positioning of condensin at centromeres is consistent with the previously demonstrated role of condensin in regulating centromere rigidity [12] , [33] , [34] . 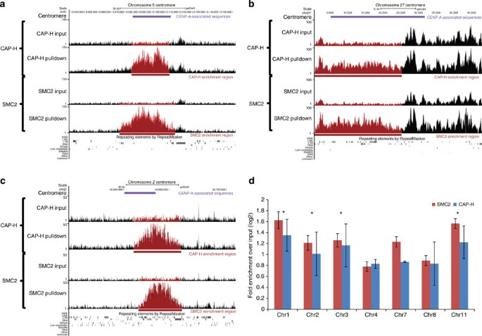Figure 3: Condensin I is densely bound at the centromeric sequences in chicken DT40 cells. (a–c) SMC2 and CAP-H pulldown enrichment to the input in the CENP-A-associated sequences (centromeres; marked in violet) in (a) chromosome 5, (b) chromosome 27 and (c) chromosome Z of chicken DT40 in a UCSC genome browser view. The coordinates of the known centromeres are chr5:3,075,314-3,104,608 and chr27:4,623-31,524 and chrZ:42,605,339-42,634,855 in galGal4 (ref.32). The centromere sequences are indicated at the top of each genome browser view. (d) Analysis of SMC2 and CAP-H enrichment to input in each consensus centromere repeat sequences derived from the chicken chromosome 1, 2, 3, 4, 7, 8 and 11 (ref.32). Error bars indicate standard errors.P-values were 4.70 × 10−3, 4.88 × 10−2, 1.50 × 10−2and 5.99 × 10−3for chromosome 1, 2, 3 and 11 (denoted by asterisk;n=5 as for both SMC2 and CAP-H).P-values were calculated using edgeR exact test with Benjamini–Hochberg FDR adjustment31. Figure 3: Condensin I is densely bound at the centromeric sequences in chicken DT40 cells. ( a – c ) SMC2 and CAP-H pulldown enrichment to the input in the CENP-A-associated sequences (centromeres; marked in violet) in ( a ) chromosome 5, ( b ) chromosome 27 and ( c ) chromosome Z of chicken DT40 in a UCSC genome browser view. The coordinates of the known centromeres are chr5:3,075,314-3,104,608 and chr27:4,623-31,524 and chrZ:42,605,339-42,634,855 in galGal4 (ref. 32 ). The centromere sequences are indicated at the top of each genome browser view. ( d ) Analysis of SMC2 and CAP-H enrichment to input in each consensus centromere repeat sequences derived from the chicken chromosome 1, 2, 3, 4, 7, 8 and 11 (ref. 32 ). Error bars indicate standard errors. P -values were 4.70 × 10 −3 , 4.88 × 10 −2 , 1.50 × 10 −2 and 5.99 × 10 −3 for chromosome 1, 2, 3 and 11 (denoted by asterisk; n =5 as for both SMC2 and CAP-H). P -values were calculated using edgeR exact test with Benjamini–Hochberg FDR adjustment [31] . Full size image Other CENP-A-associated sequences from chromosomes with repeat-rich centromeres were also tested for condensin enrichment. This analysis included centromere repeat sequences from chromosomes 1, 2, 3, 4, 7, 8 and 11, on which it is not possible to map the CENP-A distribution precisely [32] . This analysis revealed some SMC2 and CAP-H enrichment for all centromeres and significant enrichment of up to threefold over their matching input for chromosomes 1, 2, 3 and 11 ( Fig. 3d ). These results suggest that condensin may be enriched at all centromeres in DT40 cells; however, it is important to note that these repeats also occur elsewhere in the chicken genome. Condensin enrichment on the chicken centromere is also reflected using cytological methods. Immunofluorescence analysis show that both SMC2 and CAP-H are enriched at the primary constrictions of chromosomes in chicken DT40 cells ( Supplementary Fig. S8B ). Condensin I enrichment on telomeres We extended our mapping to include all major families of repetitive DNA in the chicken genome. In order to minimize artefacts due to mapping bias, we analysed condensin enrichment in two different ways: Repbase-based analysis using consensus repetitive sequences obtained from the Genetic Information Research Institute (GIRI) as a reference genome and genome-wide analysis using RepeatMasker annotations from the UCSC table browser [29] . In these analyses, we included duplicate sequences considering the nature of repetitive sequences. Overall, this analysis confirmed the preferential association of condensin with regions of high GC content ( Supplementary Figs S9 and S10 ). The Repbase analysis revealed a striking enrichment of condensin I on the telomere repeat (TTAGGG) n ( Supplementary Fig. S9 ). This enrichment of condensin I on telomere repeat sequences was also detected in our genome-wide repeat analysis ( Supplementary Fig. S10 ). Condensin I enrichment on telomeric sequences was also observed when all hexamer combinations of pulldown and input sequences were analysed for SMC2 and CAP-H ( Supplementary Fig. S11 ). A moderate enrichment of condensin I subunits was also evident on subtelomeric repeats ( Supplementary Fig. S12 ). In this, the distribution of condensin is reminiscent of that of another SMC protein complex, cohesin, which was recently shown to be enriched in subtelomeric regions [35] . Importantly, chicken repeat 1 (CR1), which comprises the largest portion of retrotransposons and also accounts for the greatest proportion of repeats in the chicken genome, does not display significant condensin I enrichment. Indeed, the longer CR1 elements exhibit less condensin binding than short fragments ( Supplementary Fig. S13 ). Validation of condensin I-binding sites Both molecular and cytological approaches confirmed our mapping of condensin I binding sites ( Figs 4 , 5 ). Quantitative PCR (qPCR) analysis of CAP-H-associated DNA (blue, n =8) using primers for selected tRNA genes at CpG islands displayed a striking enrichment of up to sixfold compared with control regions lacking condensin-associated sequence tags ( Fig. 4a ). CAP-H was also up to fourfold enriched on tRNA genes without CpG islands and on CpG islands lacking tRNA genes ( Fig. 4b,c ). Several histone genes that showed a preferential association with both SMC2 and CAP-H in our computational analysis also showed moderate-to-high enrichment in the pulldowns by qPCR analysis ( Fig. 4d ). To eliminate the possibility that DNA non-specifically bound to either the tag (SBP) or beads we generated a DT40 cell line expressing only GFP–SBP, and showed that no enrichment was observed at multiple condensin enriched sites following SBP pulldown ( Fig. 4 green, n =3, Supplementary Fig. S14 ). 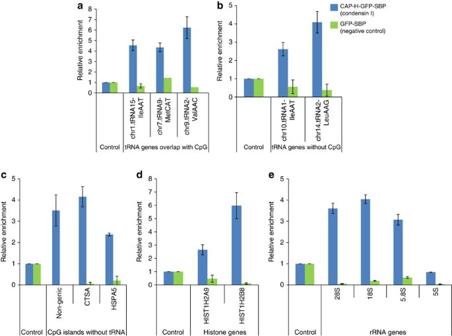Figure 4: Verification of condensin I enrichment using molecular methods in chicken DT40 cells. (a–e) Quantitative PCR was used to validate the selected condensin I enrichment regions including (a) tRNA genes overlapping with CpG islands, (b) tRNA genes without CpG island overlap, (c) CpG islands without tRNA gene overlap, (d) histone genes and (e) rRNA sequences in the CAP-H pulldown DNA (n=8 for each region; blue). Theyaxis expresses the enrichment changes from input to pulldown of the selected regions relative to that of the control. Eight independent affinity purifications using CAP-H–GFP–SBP were performed and the average quantity was normalized with respect to the control. CAP-H was enriched highly in all these selected regions in the tRNA, 28S and 18S rRNA genes, CpG islands and the histone genes. In contrast, enrichment was not observed in those selected regions in the negative control pulldown from DT40 cells expressing GFP-SBP tag only (n=3 for each region; green), supporting condensin I binding in these regions. The control sequence showed no enrichment for condensin based on our sequencing profiles (chr11:13,498,471-13,498,576 of galGal4), and therefore is not expected to show any enrichment in qPCR. The error bars indicate standard error. Figure 4: Verification of condensin I enrichment using molecular methods in chicken DT40 cells. ( a–e ) Quantitative PCR was used to validate the selected condensin I enrichment regions including ( a ) tRNA genes overlapping with CpG islands, ( b ) tRNA genes without CpG island overlap, ( c ) CpG islands without tRNA gene overlap, ( d ) histone genes and ( e ) rRNA sequences in the CAP-H pulldown DNA ( n =8 for each region; blue). The y axis expresses the enrichment changes from input to pulldown of the selected regions relative to that of the control. Eight independent affinity purifications using CAP-H–GFP–SBP were performed and the average quantity was normalized with respect to the control. CAP-H was enriched highly in all these selected regions in the tRNA, 28S and 18S rRNA genes, CpG islands and the histone genes. In contrast, enrichment was not observed in those selected regions in the negative control pulldown from DT40 cells expressing GFP-SBP tag only ( n =3 for each region; green), supporting condensin I binding in these regions. The control sequence showed no enrichment for condensin based on our sequencing profiles (chr11:13,498,471-13,498,576 of galGal4), and therefore is not expected to show any enrichment in qPCR. The error bars indicate standard error. 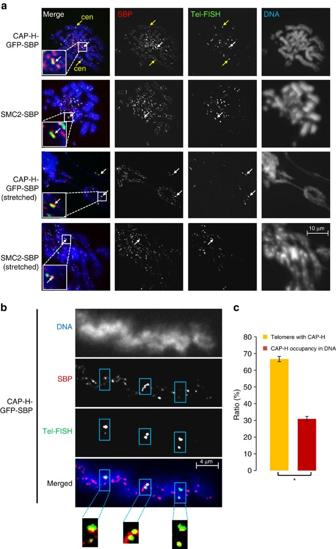Figure 5: Cytological validation of SMC2 and CAP-H enrichment at telomere repeats. (a) Telomere-FISH probes (green) and immunostaining for SMC2 or CAP-H SBP-tagged proteins (red) in both non-stretched and stretched mitotic chromosomes in chicken DT40 cells. DNA is co-stained with DAPI. The overlap of the FISH probe (telomere) and SBP signals (SMC2 or CAP-H) are indicated by a white arrow in both non-stretched (top two panels) and stretched chromosomes (bottom two panels). Their signal is also detected in the centromeric regions (primary constrictions of large chromosomes) in CAP-H–GFP–SBP cells (yellow arrow). (b) An example of chromosome telomere sequences colocalized with condensin I (CAP-H–GFP–SBP) on chromosome 1 that was used for quantification in (c). Note chromosome 1 has prominent interstitial telomere enrichment36. Chromosomes were selected that had slightly stretched CAP-H–SBP (red) and therefore discontinuous signal, thereby minimizing the chance of random overlap. For scoring, all seven macro avian chromosomes from interstitial and canonical telomere-CAP-H overlapped regions were analysed, with both regions showing a very high overlap of CAP-H and telomere signal. The scale bar is 4 μm. (c) Quantification of telomere and CAP-H overlap in mitotic DT40 cells. Approximately 67% of telomere-FISH overlaps with SBP (CAP-H). This contrasts to 31% of SBP occupancy in DNA (representing the chance of SBP overlapping with random DNA). Telomere, CAP-H and DNA signals were calculated from chromosomes from 43 separate cells (n=43). TheP-value of 1.29 × 10−7is seen using Pearson’sχ2test comparing CAP-H and telomere overlap against CAP-H occupancy in the DNA (denoted by asterisk). Full size image Figure 5: Cytological validation of SMC2 and CAP-H enrichment at telomere repeats. ( a ) Telomere-FISH probes (green) and immunostaining for SMC2 or CAP-H SBP-tagged proteins (red) in both non-stretched and stretched mitotic chromosomes in chicken DT40 cells. DNA is co-stained with DAPI. The overlap of the FISH probe (telomere) and SBP signals (SMC2 or CAP-H) are indicated by a white arrow in both non-stretched (top two panels) and stretched chromosomes (bottom two panels). Their signal is also detected in the centromeric regions (primary constrictions of large chromosomes) in CAP-H–GFP–SBP cells (yellow arrow). ( b ) An example of chromosome telomere sequences colocalized with condensin I (CAP-H–GFP–SBP) on chromosome 1 that was used for quantification in ( c ). Note chromosome 1 has prominent interstitial telomere enrichment [36] . Chromosomes were selected that had slightly stretched CAP-H–SBP (red) and therefore discontinuous signal, thereby minimizing the chance of random overlap. For scoring, all seven macro avian chromosomes from interstitial and canonical telomere-CAP-H overlapped regions were analysed, with both regions showing a very high overlap of CAP-H and telomere signal. The scale bar is 4 μm. ( c ) Quantification of telomere and CAP-H overlap in mitotic DT40 cells. Approximately 67% of telomere-FISH overlaps with SBP (CAP-H). This contrasts to 31% of SBP occupancy in DNA (representing the chance of SBP overlapping with random DNA). Telomere, CAP-H and DNA signals were calculated from chromosomes from 43 separate cells ( n =43). The P -value of 1.29 × 10 −7 is seen using Pearson’s χ 2 test comparing CAP-H and telomere overlap against CAP-H occupancy in the DNA (denoted by asterisk). Full size image To confirm condensin I association with the repetitive rRNA genes, we designed primers using rDNA consensus sequences and compared the amplicon enrichment changes from input to pulldown DNA with that of the control. This analysis revealed a highly significant enrichment of 28S, 18S and 5.8S rDNA sequences during the ChAP-seq pulldown. Thus condensin I is enriched on these RNA polymerase I-transcribed genes ( Fig. 4e , blue). By contrast, condensin I was not enriched at 5S rRNA genes, which are transcribed by RNA polymerase III. Again, the relative enrichments for the loci tested by qPCR were positively correlated with the level of enrichment seen in the ChAP-seq analysis ( Fig. 2d ). Similar to above, qPCR on GFP–SBP pulldown also shows no enrichment in any rRNA genes ( Fig. 4e , green). We also validated condensin I enrichment at telomeres and rRNA loci using a cytological immuno-FISH approach. FISH (fluorescence in situ hybridization) probes were designed to span condensin I-enriched regions including telomeres and 18S rRNA genes. For this analysis, cells cytospun onto slides were stained for condensin I using anti-SBP antibody that recognizes the SBP attached to either CAP-H or SMC2 and subsequently probed with telomere or rDNA-FISH probes ( Fig. 5a , Supplementary Fig. S15 ). The enrichment of condensin I at telomeres observed in our ChAP-seq analysis was confirmed by the immuno-FISH experiments ( Fig. 5a ). In unstretched chromosomes, where condensin I axial staining was preserved, telomere-FISH signals frequently overlapped the axial regions both at the chromosome ends and also at interstitial telomeric sequences ( Fig. 5a ). It has long been known that telomeric sequences exist not only at chromosome ends, but also interstitially, with avian chromosomes notably displaying extended tracts of interstitial telomere sequence on several chromosomes [36] . Our own data show CAP-H and telomeric sequences also appeared to overlap near centromeres and other interstitial sites ( Fig. 5a ). This overlap was also seen for both SMC2 and CAP-H when the chromatin was stretched during sample preparation ( Fig. 5a ). We then quantitated the telomere–condensin I overlap and found a high correlation between CAP-H and telomere signal (67%, P -value=1.29 × 10 −7 from Pearson’s χ 2 test), against a background of 33% overall occupancy of CAP-H in mitotic chromosomal DNA ( Fig. 5b,c ). Immuno-FISH analysis of rDNA loci using a cloned chicken 18S rRNA probe also showed consistent overlap between FISH signals and condensin I signals on chromatin from SMC2–SBP and CAP-H–GFP–SBP-expressing cell lines ( Supplementary Fig. S15 ). The combination of quantitative PCR and immuno-FISH thus provided independent verification of our condensin I ChAP-seq map in DT40 cells. Apparent bookmarking effect of condensin I It is widely accepted that transcription ceases during mitosis [37] , but that a phenomenon referred to as bookmarking may create a positional memory so that transcription factors can rapidly reassemble at promoter sequences in G1 (ref. 25 ). Alternatively, it has been suggested that transcription factor HSF2 binding to CAP-G in mitosis recruits protein phosphatase 2A to dephosphorylate and deactivate condensin I complexes, thus promoting transcription factor binding [24] . Thus, the presence of condensin at promoters could either induce or inhibit transcription during mitotic exit. Our ChAP-seq data show that condensin I binds large numbers of promoter sequences. We hypothesized that if the bookmarking model was correct, removal of condensin might misregulate the expression of the associated genes during G1. To test this hypothesis, we performed qRT–PCR on G1 cells using our previously generated CAP-H/condensin I KO cell line [38] ( Fig. 6a,b ). These cells rapidly shut off CAP-H transcription after addition of the effector molecule, doxycycline (dox). 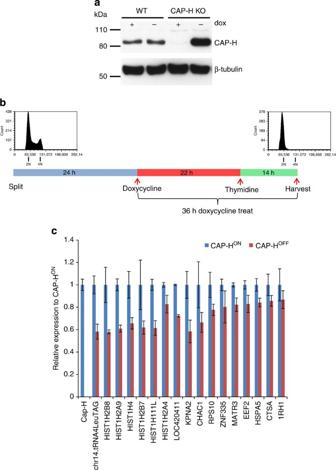Figure 6: Transcriptional analysis of condensin I/CAP-H KO cells. (a) Immunoblotting of CAP-H in CAP-H knockout and wild-type chicken DT40 cells with and without doxycycline (dox). RNAs extracted from both CAP-HONand CAP-HOFFinterphase synchronized cells using 14 h thymidine block were subjected to qRT–PCR analysis. Total time in dox for CAP-HOFF(including 14 h thymidine block) was 36 h. Immunoblotting analysis shows CAP-H is completely shut down in the knockout cells, whereas the expression of CAP-H in the wild type was not affected. This is the CAP-H depletion method applied in the qRT–PCR analysis. (b) Experimental design for the analysis, showing that CAP-H KO was dox-treated up to 36 h including 14 h thymidine block. Flow cytometry profiles show that the majority of CAP-H KO cells are in G1 phase after the thymidine block. Cells were stained in propidium iodide and analysed by FACS. The CAP-HOFFcells showed virtually no observable segregation defect at harvesting (post 36 h of dox treat)38. (c) qRT–PCR analysis of CAP-H KO cells. A total of 17 genes including one tRNA gene and six histone genes were selected for analysis based on high condensin I enrichment from our genome-wide ChAP-seq data. CAP-H transcription is also shown in this graph. Overall these genes are downregulated following CAP-H removal. The error bars indicate standard error (n=3). Figure 6: Transcriptional analysis of condensin I/CAP-H KO cells. ( a ) Immunoblotting of CAP-H in CAP-H knockout and wild-type chicken DT40 cells with and without doxycycline (dox). RNAs extracted from both CAP-H ON and CAP-H OFF interphase synchronized cells using 14 h thymidine block were subjected to qRT–PCR analysis. Total time in dox for CAP-H OFF (including 14 h thymidine block) was 36 h. Immunoblotting analysis shows CAP-H is completely shut down in the knockout cells, whereas the expression of CAP-H in the wild type was not affected. This is the CAP-H depletion method applied in the qRT–PCR analysis. ( b ) Experimental design for the analysis, showing that CAP-H KO was dox-treated up to 36 h including 14 h thymidine block. Flow cytometry profiles show that the majority of CAP-H KO cells are in G1 phase after the thymidine block. Cells were stained in propidium iodide and analysed by FACS. The CAP-H OFF cells showed virtually no observable segregation defect at harvesting (post 36 h of dox treat) [38] . ( c ) qRT–PCR analysis of CAP-H KO cells. A total of 17 genes including one tRNA gene and six histone genes were selected for analysis based on high condensin I enrichment from our genome-wide ChAP-seq data. CAP-H transcription is also shown in this graph. Overall these genes are downregulated following CAP-H removal. The error bars indicate standard error ( n =3). Full size image CAP-H ON/OFF cells were analysed for gene expression in G1 by qRT–PCR using primers specific for genes shown to be enriched for condensin I from our ChAP-seq analysis. The analysis was performed at 36 h post dox addition. At this time the CAP-H protein is efficiently depleted, but cells do not yet show obvious growth or cellular defects [38] ( Fig. 6a,b ). FACS analysis confirmed that most of the cell population was in G1. In total we analysed expression of 17 selected genes including a tRNA gene that had shown overlap with condensin I peaks at their promoters. Strikingly, all 17 showed a decrease in transcription levels during G1 following condensin I removal, consistent with a role for condensin in bookmarking genes for expression during early G1 ( Fig. 6c ). We describe here the first genome-wide map of condensin I on vertebrate mitotic chromosomes using conditional knockout cell lines in which SBP-tagged SMC2 or CAP-H provide the sole sources of bulk condensin and condensin I, respectively. Streptavidin pulldowns followed by next-generation sequencing of the affinity-purified DNA have yielded a map of the distribution of condensin I on mitotically blocked DT40 chromosomes. The pattern of condensin distribution on chromosomes shows a remarkable degree of evolutionary conservation. Most condensin was found in the promoter regions of highly transcribed genes, but condensin I enrichment was also clear on tRNA and rRNA genes and at key genomic structures essential for proper chromosome segregation including centromeres and telomeres. This vertebrate condensin map shares many features with maps previously published for the distribution of B. subtilis SMC protein [15] and for the distribution of condensin in yeast genomes [17] , [18] . This is particularly remarkable when one considers that bacteria do not package their DNA with histones, and that yeast chromosomes do not undergo visible morphological condensation during mitosis. Furthermore, in vertebrates, the condensin I complex is actually cytoplasmic during interphase. Although our analysis did not reveal any association of condensin with a single type of DNA sequence, we did observe definite patterns of condensin distribution across the genome. In yeast, condensin is enriched on tRNA and rRNA genes [17] , [18] , and the B-BOX motif of tRNA genes has been implicated in condensin recruitment [17] . This association of condensin with tRNA genes in yeast may also be promoted by physical interactions between condensin subunits SMC2 and SMC4 and RNA polymerase III and its transcription factor TFIIIC [39] . Chicken condensin exhibits a preferential association with CpG island promoters. It is also enriched over TSSs of highly expressed genes, whereas the complex is relatively depleted from the bodies of genes. Together, these results reveal that the position of condensin on mitotic chromosomes correlates strongly with patterns of gene activity. As transcription ceases during mitotic chromosome compaction and as condensin I is cytoplasmic during interphase, it is therefore unlikely that the transcriptional process itself influences this distribution of condensin on mitotic chromosomes. Instead, one possible explanation is that condensin association with chromatin regions may be affected by chromatin marks. Indeed, a previous study has linked a histone modification, H4 lysine 20 methylation, with condensin II association with chromosomes during interphase [40] . In mitotic cells, Aurora B phosphorylation of condensin I promotes its association with H2A and H2A.Z [41] , confirming the involvement of chromatin in condensin binding to chromosomes. Of course, bacterial chromosomes lack histones, but their transcription is presumably ongoing during the process of cell division, so chromatin marks might not be required to maintain the association of condensin with highly transcribed genes [15] . It has been suggested that condensin ‘bookmarks’ genes so that they can be efficiently transcribed during or shortly after mitotic exit. Our data support this role for condensin I and show that the binding correlates strongly with actively transcribed genes. It will be important to determine in future experiments whether the numerous promoter regions preferentially associated with condensin I are associated with loci that exhibit a tendency towards earlier expression during mitotic exit into G1 and, indeed, whether their expression during mitotic exit is altered by condensin I depletion. The notion of SMC proteins regulating transcription is gaining momentum with several studies linking cohesin to regulation of gene expression, notably through long-range enhancer interactions [42] . It is therefore likely that condensin might also act in trans to regulate gene expression and possibly regulate promoters not directly enriched for condensin. Of course, it remains possible that condensin ‘reads’ transcription-associated chromatin marks when establishing stable association with mitotic chromosomes, but does not actively participate in transcriptional regulation. At the simplest level, the observed binding at active promoters reflects a preference for condensin I association at open (accessible) chromatin. The non-random association of condensin I with the genome is also apparent when one examines the association of the complex with repeated DNA elements. Condensin I appears to be relatively depleted from most repeat families but it is substantially enriched on both centromeric and telomeric repeats. Condensin I binding at yeast centromeres is well documented [10] , [17] , and condensin is also enriched at the centromere-like par S locus as well as on tRNA and rRNA genes in B. subtilis [15] . Thus, these features of condensin distribution are remarkably conserved throughout evolution. In vertebrates, condensin is important for establishing the compliance (stretchiness) of the centromeric ‘spring’ that links sister kinetochores during early mitosis. Our previous studies have indicated that CENP-A chromatin is more tightly packaged and resistant to stretching than bulk chromatin [43] , [44] . The inner centromeric chromatin becomes abnormally flexible in the absence of condensin, so that kinetochores under tension from the spindle often stretch well out from the bodies of the chromosomes with centromeres showing a marked increase in inter-kinetochore distance [33] , [34] . This abnormal response to tension in the inner centromeric chromatin appears to be correlated with a delay in satisfaction of the spindle assembly checkpoint. The telomeric enrichment of condensin I has not been reported at the molecular level in any other species, although condensin does have a role in telomere segregation in S. pombe , with Cut14/SMC2 and Cut3/SMC4 mutants displaying telomere entanglement [45] . Notably, however CAP-H has been reported to overlap cytologically with telomeres during mouse male meiosis and mitosis as judged by colocalization with the telomere protein TRFI [46] . This cytological observation may be due to the large tracts of the telomere repeat in mouse [47] . Our FISH data also reveal telomere and condensin I colocalization at the chromosome ends and at interstitial telomeric sequences. Whether there is a specialized function of condensin at vertebrate telomeres remains a question for future study. A wide variety of evidence has confirmed that condensin complex(es) have an essential role in mitotic chromosome architecture. Remarkably, 20 years after the discovery of condensin, its exact mechanism of action remains enigmatic. One obvious possibility is that condensin is involved in establishing a loop-domain architecture in mitotic chromosomes [14] . Indeed, classical electron microscopy studies suggested that mitotic chromosomes are organized into ~30- to 100-kb loop domains [48] , [49] . The results of our genome-wide condensin mapping are broadly consistent with their observations. We observed an average distance between peaks of 172 kb for SMC2 (total condensin) and 257 kb for CAP-H (condensin I), taking into account the 1.2-Gb size of the haploid chicken genome. The distance between peaks for SMC2 is greater than the 90 kb estimated from proteomics experiments [50] ; however, the latter estimate assumed that condensin molecules were evenly spaced along the genome, whereas our measurements likely reflect the presence of clusters of condensin at highly enriched loci. Our data, which were confirmed using qPCR and immuno-FISH, most likely reflect the most abundant or stable condensin I sites in the chicken genome, as condensin I is relatively mobile on chromosomes [12] . Highly mobile or less-enriched sites might be beyond the detection limits of ChAP-seq analysis. Furthermore, as our analysis is on mitotically blocked cells that enrich for more condensed chromosomes. Our ChAP-seq data therefore might be under-represented in non-blocked metaphase chromosomes where condensin I could possibly occupy additional positions given the dynamic nature of the complex. However, overall our data are consistent with earlier models that condensin complexes might help to define structural domains that are essential for stable mitotic chromosome architecture. A prominent feature of our analysis is that the highest accumulation of condensin I was found at structural regions of the chromosome, including centromeres and telomeres. Significantly, both of these features display a cytological constriction, most visibly with centromeres but also seen in telomeres using FISH analysis [51] , [52] . Furthermore, secondary chromosome constrictions are observed at rRNA genes, which also exhibit a higher enrichment of condensin. In light of these observations we suggest that structural domains on the chromosome may be differentially constrained by condensin I-mediated looping ( Fig. 7 ). The higher concentration of condensin I at telomeres and centromeres may lead to the shortening of chromatin loops and thereby provide these regions with greater rigidity. 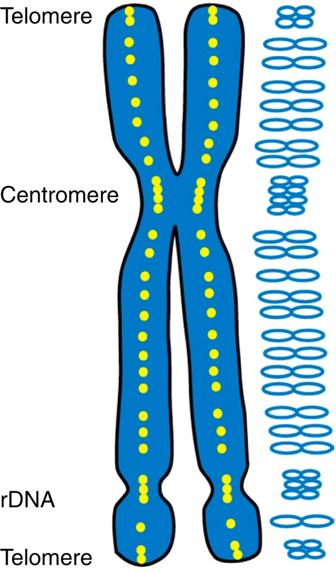Figure 7: Distribution density of condensin shapes the metaphase chromosome. The condensin complex (yellow circles) gathers the chromatin into lateral loops (blue), which are centred along a chromatid axis. Chromatin loop size determines the overall width of mitotic chromatids. Large loops are regularly spaced within and between genes to compact most of the genome into sausage-shaped chromatids. At specialized loci such as the centromeres, telomeres and rDNAs, chromatin loops are smaller, producing constricted regions. Figure 7: Distribution density of condensin shapes the metaphase chromosome. The condensin complex (yellow circles) gathers the chromatin into lateral loops (blue), which are centred along a chromatid axis. Chromatin loop size determines the overall width of mitotic chromatids. Large loops are regularly spaced within and between genes to compact most of the genome into sausage-shaped chromatids. At specialized loci such as the centromeres, telomeres and rDNAs, chromatin loops are smaller, producing constricted regions. Full size image Our most surprising result is that the distribution of condensin I in the chicken genome is so reminiscent of the distribution of condensin in B. subtilis [15] and in the budding yeast [17] , [18] . This suggests that condensin must have roles that are independent of the packaging of the DNA into chromatin and chromosome condensation during mitosis. One possibility is that condensin’s ability to supercoil DNA [53] may be important for gene regulation–for example in gene bookmarking. The analysis reported here has created an important resource that not only may explain some of condensin’s known functions but also encourages new avenues of research as we search for a common role for condensin across the three kingdoms of life where its distribution has been mapped. Cell culture and synchronization Chicken lymphoma B DT40 cell culture was performed as previously described [9] , [54] . SBP-tagged SMC2 or CAP-H rescue cell lines were cultured in 200 ng ml −1 doxycycline (dox). Repression of the tetracycline-repressible CAP-H gene was induced by addition of 100 ng ml −1 dox for 36 h for qRT–PCR [38] . For synchronizing chicken DT40 cells in mitosis, cells were blocked in 500 ng ml −1 nocodazole for 13–14 h as described previously [50] , resulting in a mitotic index of at least 80%. The mitotic index was calculated by both counting cells with the NEBD and flow cytometic analysis with anti-MPM2 mitotic marker staining (Millipore). For synchronizing the DT40 cells in G1 phase, the cells were blocked in 4 mM thymidine for 13–14 h. Chromatin Affinity Purification-sequencing (ChAP-seq) ChAP-seq was performed using chromatin affinity purification method as previously described [55] . In brief, 3 × 10 8 DT40 cells with SBP-tagged SMC2 and CAP-H transgene rescuing the knockout background [38] , [54] were fixed in 1% formaldehyde (Merck) for 5 min and the crosslinking was stopped in 125 mM glycine. The crosslinked cells were lysed in 1 ml lysis buffer (0.5% ( w / v ) SDS, 100 mM EDTA, 50 mM Tris/HCl (pH 7.4), 30 mg ml −1 RNase A and freshly added protease inhibitors (Roche)). The chromatin in the crude lysate was sheared to 100–500 bp by sonication (Covaris) and the supernatant was subjected to affinity purification using streptavidin-resin beads (Pierce) resuspended in 10 ml binding buffer (50 mM Tris/HCl (pH 7.4), 250 mM NaCl, 0.5% ( v / v ) NP-40, 0.1% ( w / v ) deoxycholate and freshly added protease inhibitors (Roche)) for 2 h at 4 °C. Streptavidin-bound protein-DNA was natively eluted in 0.5 ml elution buffer (50 mM Tris/HCl (pH 7.4), 250 mM NaCl, 0.5% ( v / v ) NP-40, 0.1% ( w / v ) deoxycholate, 4 mM biotin) at 4 °C for 1 h following several washing steps. The eluates were reversely crosslinked at 65 °C overnight with protein digestion in 1 mg ml −1 proteinase K (Roche), followed by DNA extraction using phenol/chloroform and ethanol precipitation. The precipitated DNA was resuspended in TE buffer (10 mM Tris-Cl (pH 7.5), 1 mM EDTA) and subjected to the Illumina sequencing with 12 million 50-bp single-end reads per sample, which allows 50% of the haploid chicken genome coverage. Such coverage is thought to be sufficient according to previous studies [40] , [56] . Glycogen (4% ( v / v ); Roche) was used as a carrier during the DNA precipitation. ChAP-seq data analysis The sequence reads from the Illumina Hiseq 2000 sequencing were aligned to the latest chicken genome (galGal4) obtained from UCSC table browser following the quality control by FASTQC [57] . Primary alignment analysis was performed using Burrows–Wheeler Aligner (BWA) v0.5.8 (ref. 58 ) with default mapping parameters for all the data analysis in this study. Additional mapping was performed using Bowtie v0.12.7 (ref. 59 ) with default mapping parameters to confirm the data reproducibility. The output data were converted to BAM using Samtools for further analysis [60] . The total numbers of sequence tags aligned using BWA are shown in Supplementary Table S1 . The duplicate sequences were removed using SAMtools v0.1.8 (ref. 60 ) before further analyses except for the repetitive sequence analysis (see below). The enrichment regions of the pulldown sequences of SMC2/CAP-H, also referred as peaks, were identified using MACS v1.4.1 (ref. 26 ). The parameters used for peak calling includes the chicken reference genome size as 1,016 Mb (excluding the repetitive sequences from the original chicken genome size 1.2-Gb), tag size as 49 bp and band width as 200 bp; other parameters remained default. As major peaks were consistent between each replicate, pulldown DNA sequences were pooled in order to increase the DNA coverage before peak calling. Respective input sequences were scaled to the size of the pooled pulldown sequence data for unbiased analysis. The number of regions that overlap between SMC2 and CAP-H peaks were identified using Bioconductor v2.3 package ChIPpeakAnno v2.8.0 (ref. 61 ). For peak distribution analysis, the number of peaks landing in each genomic feature including promoters, genes (including 5′UTR, coding exons, introns and 3′UTR of RefSeq genes) and extragenic were counted. We defined promoters as 2 kb upstream of TSSs of all RefSeq genes in the galGal4 chicken genome. The coordinates of the RefSeq genes were obtained from the NCBI [27] . The genomic distribution of each feature was calculated as their base-coverage in the total chicken genome. Gene ontology analysis Gene ontology analysis was performed on a list of genes overlapping with both SMC2 and CAP-H peaks and CpG islands using DAVID/EASE [62] . Non-coding RNA gene analysis The coordinates of the tRNA genes in galGal4 were obtained from the Genomic tRNA database ( gtrnadb.ucsc.edu ) [28] , and the enrichment of pulldown sequence tags mapped to all 279 tRNA genes were calculated using bedtools [63] . Duplicate sequence tags were removed to prevent PCR amplification bias. If no input sequences were counted in a region for an experiment, the average number of input sequence tags aligned in the feature was used for enrichment calculation. Venn Diagrams ( Fig. 2a ) showing the tRNA genes having more than twofold enrichment over the input from this analysis were generated using Cistrome integrative analysis tools [64] . rRNA coordinates were extracted from the RepeatMasker table from the UCSC table browser and calculated as described above. The pooled pulldown sequences mapped to the galGal4 genome were used for this analysis. Duplicate sequence tags were retained in this analysis. Pulldown sequences were aligned to each type of rRNA gene consensus sequence obtained from GenBank as reference genome using BWA with default parameters and the numbers of aligned sequences were calculated using SAMtools. Each set of replicate sequence data was independently used for this analysis. Repetitive sequence analysis In order to prevent mapping bias, the pulldown enrichment in repetitive sequences were analysed in two ways: using genome-wide RepeatMasker annotation of the chicken genome from UCSC table browser [65] or using the consensus sequences of each type of repetitive sequences called Repbase from Genetic Information Research Institute (GIRI; www.girinst.org ) [29] . The duplicate sequences were retained for this analysis due to the nature of repetitive sequences appearing in multiple locations in the genome. For genome-wide analysis, bedtools was used to count sequence tags overlapping each annotation of RepeatMasker [63] . For Repbase analysis, the pulldown and input DNA sequences were aligned to the Repbase sequences using BWA with default parameters, and the aligned sequence read numbers on each type of the consensus sequence were counted using SAMtools for pulldown enrichments and coverage analysis. TSS analysis Sequence alignment data in BAM format were transformed into BED format using bedtools and used for sequence density analysis at TSSs with EpiChip v0.9.7 (ref. 66 ). Default parameters were used. Duplicate sequence tags were removed using SAMtools [60] before performing this analysis. All RefSeq annotated gene TSS coordinates were obtained from NCBI [27] . Accession numbers of sequence data A number of the sequences were obtained from GenBank/DDBJ/EMBL in this study for condensin enrichment in centromere and rRNA gene sequences. Accession numbers of the rRNA sequences includes FM165415.2, AF173612.1, DQ018753.1, AF419701.3, AF419700.1 for 28S, 18S, and 5.8S intergenic spacer, 5S intergenic spacer, and 5S rRNA genes, respectively. Centromere sequences accession numbers include: AB556722.1, AB556723.1, AB556724.1, AB556725.1, AB556726.1, AB556727.1, AB556728.1 for centromere sequences of chromosome 1, 2, 3, 4, 7, 8, 11, respectively. Accession numbers of the fully sequenced centromeres of chromosome 5, 27, Z are AB556729.1, AB556730.1, AB556731.1, respectively. For transcription level analysis between condensin-bound and unbound genes, two independent Affymetrix array data of wild-type DT40 cells (GSM210532 and GSM465893) were obtained from Genome Expression Omnibus (GEO). Statistical analysis of pulldown enrichment We calculated the significance of the enrichment of each replicate pulldown compared with the input samples in some analysis (for example, rRNA genes and centromere; Figs 2d and 3d and Supplementary Fig. S8 ) using the Bioconductor v2.3 package edgeR v.3.2.3 (ref. 31 ). EdgeR uses empirical Bayes estimation and exact tests based on the negative binomial distribution to perform differential signal analysis of genome-scale count data. We calculated differential enrichment of the pulldown versus input using the edgeR exact test with tag-wise dispersion estimation. P -values were corrected for false discovery rate using the Benjamini–Hochberg method [31] . The significant difference between two groups (for example, transcription between condensin-bound and unbound genes ( Fig. 1c ), tRNA genes with and without CpG islands ( Fig. 2c ), comparison between subtelomere and other satellite sequences ( Supplementary Fig. S12 )) were calculated using the Wilcoxon Rank Sum test, which is appropriate for comparing two groups with different sample sizes. In order to show that the overlap between condensin (CAP-H–GFP–SBP) and telomere-FISH is not by chance, χ 2 test was applied ( Fig. 5c ). The proportions of telomere-FISH signals overlapping with CAP-H were counted and the proportions of CAP-H signal occupancy in DNA (representing the probability of condensin binding to any part of chromatin) were measured using ImageJ, and these two data sets were analysed using Pearson’s χ 2 test. Silver staining The pulldown eluents from the chromatin affinity purification were boiled in SDS-sample buffer (Life Technology) at 95 °C for 5 min and subjected to SDS–PAGE on 4–12% BisTris gels (Life Technologies), followed by silver staining as previously described [67] . The gel was fixed in fixing solution (50% ( v / v ) methanol, 12.5% (v/v) acetic acid and 0.05% ( v / v ) formaldehyde) for 30 min, followed by two washing steps in washing solution (30% ( v / v ) ethanol). Following sensitization of the gel in 0.02% ( w / v ) sodium thiosulfate and hydration, the gel was silver-stained in the silver staining solution (0.2% ( w / v ) silver nitrate and 0.076% ( v / v ) formaldehyde) for 30 min, followed by developing in developing solution (10% ( w / v ) sodium carbonate, 0.1% ( v / v ) formaldehyde and 0.001% ( w / v ) sodium thiosulfate). Developing was stopped with incubation in the fixing solution. Immuno-FISH 18S rRNA gene probe primers were designed to the complete 18S ribosomal RNA gene, GenBank accession number, AF173612 ; primer sequences: 18Sgg-f ATTAAGCCATGCATGTCTAAGTAC and 18Sgg-r CTTCCTCTAGATAGTCAAGTTCG. The product size was 1,733 bp. The DNA fragment was amplified using standard PCR conditions, purified and then cloned into pGEM-T-easy (Promega). A telomere (TTAGGG) n probe, plasmid htel/neo was used for immuno-FISH. The 18S rRNA and telomere probes were labelled with DIG or biotin for use as a FISH probe after nick translation using standard protocols. Immuno-FISH was performed according to standard protocols [68] . Briefly, 1 h nocodazole-blocked CAP-H–SBP and SMC2–SBP cells were hypotonically swollen and cytospun onto slides and the resulting stretched chromatin was co-stained with anti-SBP (1/200) and labelled with 18S rRNA or telomere probes. The cytospin process produced both stretched and unstretched chromosomes and representatives of each were displayed in the figures. Immunoblotting analysis Wild type (WT) and SMC2–SBP or CAP-H–GFP–SBP DT40 cell lines were lysed in lysis buffer (50 mM Tris/HCl (pH 7.4), 250 mM NaCl, 0.5% ( v / v ) NP-40, 30 μg ml −1 RNase A and freshly added protease inhibitors (Roche)), followed by sonication using the Bioruptor (Diagenode). Equal amounts of protein from crude lysate were run on 4–12% BisTris gels (Life Technologies) and immunoblotted as described previously [55] . The blots for both WT and SBP-tagged SMC2 or CAP-H were probed with rabbit anti-SMC2 or rabbit anti-CAP-H antibodies, respectively, both at 1:2,500 in 1% ( w / v ) bovine serum albumin (BSA) PBS/ 0.2% ( w / v ) Tween20 (PBST) for 2 h, followed by anti-rabbit horseradish peroxidase staining (Millipore) at 1:60,000 in PBST for 2 h. The blots were analysed using a chemiluminescence kit (GE Healthcare). Flow cytometry DT40 cells were washed in PBS and homogenized, followed by fixation in 70% ethanol at 4 °C overnight. For cell cycle analysis, cells were washed three times in PBS and either stained in propidium iodide (Sigma) for 5 min at room temperature or immunostained using mouse anti-MPM2 antibody (Millipore) for 1 h followed by donkey anti-mouse Alexa-488 antibody (Life Technologies) staining for 30 min at room temperature. For apoptosis analysis, annexin 5-PE-Cy5 (Bio Vision, Inc) was applied according to the manufacturer’s instruction. All assays were analysed using FACSCalibur (Becton Dickinson) and CellQuest (Becton Dickinson). Quantitative PCR The purified DNA was analysed by qPCR using 7900HT Fast Real-Time PCR System machine (Life Technology) and FAST SYBR Green Master Mix (Life Technology). Primers are designed specifically for regions tested including tRNA genes and rRNA genes as well as negative control, and their sequences are available in Supplementary Table S3 . The assay was performed on eight and three independent pulldown samples from CAP-H–GFP–SBP and GFP–SBP (tag only) affinity purification, respectively, for each primer pair. Quantitative RT–PCR analysis Total RNAs were extracted from both CAP-H ON and CAP-H OFF cells blocked in interphase by 4 mM thymidine using a mir Vana miRNA Isolation Kit (Ambion) according to the manufacturer’s instruction. Residual DNA was removed using TURBO DNA-free Kit (Ambion). Total RNA (2 μg) from each sample was reverse-transcribed with High Capacity cDNA Reverse Transcription Kits (Applied Biosystems) according to the manufacturer’s protocols. All cDNA samples were diluted to 15 ng μl −1 for qRT–PCR analysis. qRT–PCR was performed to examine the relative quantification of the expression level of selected genes based on the ChAP-seq. cDNA (15 ng) of each sample was amplified using SYBR Green PCR Master Mix (Applied Biosystems) according to the manufacturer’s protocol. Primers used in this experiment are available in Supplementary Table S4 . The reaction was carried out in optical 384-well standard plates (Applied Biosystems) using HT9600 Fast real-time PCR system (Applied Biosystems). The relative quantification of the selected gene expression was calculated using 2 − ΔΔCt method after the threshold cycle ( Ct ) was normalized with the Ct of CENP-C . To ensure accuracy, at least three different experiments were performed individually and each sample was run in triplicates. Deposition of data : Raw and processed data from this study have been deposited in the NCBI Gene Expression Omnibus under accession number GSE45552 . How to cite this article: Kim, J. H. et al . Condensin I associates with structural and gene regulatory regions in vertebrate chromosomes. Nat. Commun. 4:2537 doi: 10.1038/ncomms3537 (2013).